Dissecting the mammary gland one cell at a time 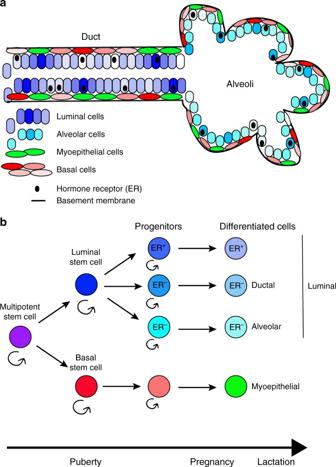Fig. 1 Simplistic model of mammary epithelial cell differentiation hierarchy.aSchematic outline of a ductal-alveolar unit with location of the various cell types indicated.bA putative map of mammary epithelial cell differentiation. A multipotent stem cell present during development gives rise to luminal epithelial and basal stem cells, which further divide into luminal and basal progenitors during puberty. Ductal and alveolar hormone-receptor negative progenitors are distinct lineages and there is also a separate hormone receptor positive luminal lineage Dissecting cellular differentiation hierarchies in the mammary gland is a prerequisite for understanding both normal development and malignant transformation during tumorigenesis and tumor cell-of-origin. To achieve these goals, several recent papers utilized single cell RNA-seq and lineage tracing to improve our understanding of the composition of the mammary epithelium at different developmental stages.